GWAS identifies four novel eosinophilic esophagitis loci Eosinophilic esophagitis (EoE) is an allergic disorder characterized by infiltration of the oesophagus with eosinophils. We had previously reported association of the TSLP/WDR36 locus with EoE. Here we report genome-wide significant associations at four additional loci; c11orf30 and STAT6 , which have been previously associated with both atopic and autoimmune diseases, and two EoE-specific loci, ANKRD27 that regulates the trafficking of melanogenic enzymes to epidermal melanocytes and CAPN14 , that encodes a calpain whose expression is highly enriched in the oesophagus. The identification of five EoE loci, not only expands our aetiological understanding of the disease but may also represent new therapeutic targets to treat the most debilitating aspect of EoE, oesophageal inflammation and remodelling. Eosinophilic esophagitis (EoE OMIM 610247) is an inflammatory disorder of the oesophagus, histologically characterized by accumulation of eosinophils in the oesophageal epithelium. Clinical symptoms of EoE include dysphagia, failure to thrive, vomiting and epigastric or chest pain. A diagnosis of EoE is made following endoscopy and biopsy on finding isolated eosinophils in the oesophagus having ruled out gastro-oesophageal reflux [1] . Multiple reports indicate a gender bias, with males predominantly affected [2] . The rate of co-existing atopic disease in other organs is high, with up to 70% of the subjects presenting with asthma or atopic dermatitis [2] . EoE is considered a food allergy-related disorder based on the high rate of food allergen sensitization and a higher rate of food anaphylaxis in cases compared with the general population [1] , [3] . Furthermore, the majority of EoE cases undergo disease remission following introduction of an elemental formula diet that lacks allergens. Experimental modelling of EoE in mice has demonstrated a key role for adaptive immunity and Th2-cell cytokines (especially interleukin (IL)-5 and -13) in the disease process and a strong connection between allergic sensitization and inflammation in the respiratory tract and skin [4] . The stringent diagnostic criteria for EoE, that include biopsy-proven eosinophilic infiltration of the oesophagus, result in a phenotypically homogenous case series that is well powered for genome-wide association study (GWAS) and a potentially powerful model to study the genetics of food allergy and atopy in general. Increasing evidence suggests a strong genetic component to EoE [5] . In a pediatric study, nearly 10% of the parents of EoE patients had a history of oesophageal strictures and ~8% had biopsy-proven EoE [5] , [6] . However, there has only been one replicated locus identified to date. Using a GWAS approach, we have previously reported genome-wide association of multiple variants at the thymic stromal lymphopoetin ( TSLP ) locus in a cohort of EoE patients [7] . Here we report the results of an expanded GWAS totalling 936 cases and 4,312 controls in an imputed data set that included ~2.3 M variants, identifying four novel EoE associated loci. EoE GWAS The data set was split into discovery and replication sets based on the Illumina arrays on which the samples were genotyped (HH550/HH610 or OmniExpress). Following GWAS of the discovery cohort ( n =603 cases and 3,637 controls) by logistic regression of the binary EoE phenotype adjusting for sex and the first 10 eigenvectors of the principal component analysis, five loci remained genome-wide significant (cut-off P ≤5 × 10 −8 ) following multiple testing correction ( Fig. 1 , Supplementary Fig. 1 ). The same variants at the TSLP , c110rf30 and CAPN14 loci were also associated with EoE in the replication cohort ( n =333 cases and 675 controls). 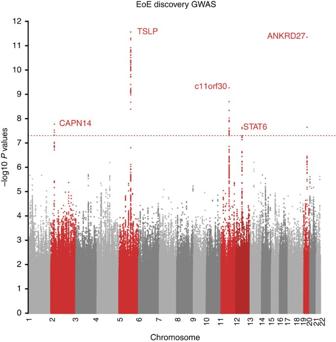Figure 1: Manhattan plot of the EoE discovery GWAS. n=603 cases and 3,637 controls. −log10Pvalues on theyaxis plotted against ascending physical position on thexaxis. The dotted red line represents the genome-wide significance thresholdPvalues ≥5 × 10−8. The genome-wide significant variants mapped to the previously reported TSLP locus [7] (top single nucleotide polymorphism (SNP) discovery cohort rs1438673; P 1.74 × 10 −12 , odds ratio (OR) 0.62; P replication 3.84 × 10 −3 , OR replication 0.792; P combined 1.5 × 10 −13 , OR 0.67; Supplementary Table 1 , Supplementary Fig. 2 ) a novel locus on chr11q13.5 that contains the c11orf30 gene (top SNP rs55646091; P discovery 5.83 × 10 −10 , OR 2.21; P replication 4.33 × 10 −3 , OR replication 1.584; P combined 7.67 × 10 −11 , OR 2.41; Supplementary Table 1 ) and a novel locus on chr2p23.1 that spans the CAPN14 gene (top SNP rs74732520; P discovery 1.69 × 10 −8 , OR 1.78; P replication 5.86 × 10 −3 , OR replication 1.56; P combined 4.16 × 10 −9 , OR 1.91; Supplementary Table 1 , Supplementary Fig. 4 ). Two further novel loci surpassed genome-wide significance in the discovery cohort that we were not sufficiently powered to replicate, a locus on chr12q13.3 that spans the STAT6 gene (top SNP rs167769, P discovery 2.29 × 10 −8 , OR 1.49; Supplementary Fig. 5 ) and a locus on chr19q13.11 spanning the ANKRD27 gene (top SNP rs3815700, P discovery 4.54 × 10 −12 , OR 1.65; Supplementary Fig. 6 ). Meta-analysis of the discovery and replication cohorts did not identify any additional genome-wide significant loci, however, a sixth intergenic locus upstream of NOVA1 at chr14q12 showed a trend towards association (top SNP rs8008716, P combined 6.9 × 10 −8 , OR 1.71; P discovery 2.07 × 10 −6 , OR 1.45; P replication 2.2 × 10 −3 , OR 1.57). To determine if the c11orf30 and STAT6 signals were driven by the high rates of EoE comorbidities we carried out conditional analyses at the two loci, including asthma, atopic dermatitis and allergic rhinitis status as a covariate for the c11orf30 locus and sensitization as a covariate at the STAT6 locus in a subset of 265 cases for which we had individual-level comorbidity data. 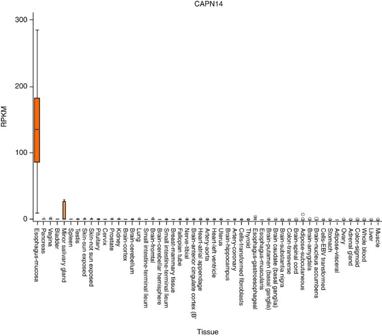Figure 2: CAPN14 is highly expressed in the oesophagus. Transcriptome-sequencing data from the GTEx project indicates CAPN14 is predominantly expressed in the oesophageal mucosa (n=106). Each boxplot represents a measure of CAPN14 gene expression, plotted on theyaxis for a given tissue, plotted on thexaxis. The measure of expression used is reads per kilobase million (RPKM). The boxplot whiskers represent the data range across the 106 replicates, with the notch in the box representing the median expression value. Residual association with EoE was detected at both loci following the conditional analyses ( Supplementary Table 2 ). Figure 1: Manhattan plot of the EoE discovery GWAS. n =603 cases and 3,637 controls. −log10 P values on the y axis plotted against ascending physical position on the x axis. The dotted red line represents the genome-wide significance threshold P values ≥5 × 10 −8 . Full size image The linkage disequilibrium patterns between the associated variants at the c11orf30 locus indicated the presence of independent effects ( Supplementary Fig. 3 ). Conditional analyses in the discovery cohort on the top SNP, rs55646091, confirmed the existence of an independent effect, tagged by the rs11236791 variant, at the locus ( Supplementary Table 3 ). Oesophageal biopsy transcriptome sequencing RNAseq of primary epithelial cells derived from oesophageal biopsy of nine EoE patients and three controls confirmed expression of TSLP , c11orf30, CAPN14, STAT6, ANKRD27 and NOVA1 in oesophageal epithelial cells. We detected expression of 12,407 genes out of an estimated 21,000 (ref. 8 ). Examining differential expression between cases and controls, CAPN14 expression was almost fourfold increased in EoE cases compared with controls (cases FPKM 9.82807, control FPKM 0.630785; log2 (fold change) 3.96169; P 5 × 10 −5 ; Supplementary Table 4 ). The remaining four genes showed subtle, albeit not statistically significant expression level changes. Examining other genes at the association loci, expression of both WDR36 and GALNT14 was detected but without any significant differences in cases and controls. LRRC32 was not expressed at appreciable levels ( Supplementary Table 4 ). Pathway analysis of the differentially expressed genes in cases and controls from the transcriptome-sequencing experiment indicated an enrichment of cell cycle-related gene ontology (GO) terms amongst genes whose expression was decreased in cases versus controls and an enrichment of epidermis and epithelial cell development and differentiation GO terms in the list of gene whose expression increased in cases versus controls ( Supplementary Table 5 ). Since our initial report of association of TSLP variants with EoE in under 200 patients, TSLP has been associated with allergic sensitization [9] , [10] , asthma [11] , [12] and allergic rhinitis [13] in GWAS that required thousands of cases to achieve significance. Variants at the c11orf30 locus have been associated with seasonal allergic rhinitis [13] , ulcerative colitis [14] , Crohn’s disease [15] , atopic dermatitis [16] , [17] , asthma [18] and allergic sensitization [10] , albeit with much lower ORs (range 1.09 in asthma to 1.22 in atopic dermatitis). Asthma, atopic dermatitis and allergic rhinitis are common comorbidities of EoE. We therefore carried out a conditional analysis on asthma, atopic dermatitis and allergic rhinitis status in the EoE cases demonstrating that the observed c11orf30 association with EoE was independent of comorbidity status. The c11orf30 gene encodes, EMSY, a transcriptional regulator that was initially identified as a BRCA-2-associated protein that is amplified in human mammary adenocarcinomas [19] . More recently, EMSY has been identified as a central component in a novel Akt-dependent mechanism by which interferon and other growth factors regulate the expression of interferon-stimulated genes [20] . STAT6 is a key player in the IL-4 pathway. STAT6 when activated by IL-4, through its receptor IL-4R, controls the expression of GATA3, the Th2 master regulatory transcription factor, as well as the IL-4 locus control region [21] . STAT6 has been associated with serum IgE levels [22] and allergic sensitization [10] , through GWAS. Conditional analysis at the STAT6 locus on sensitization status indicated the observed association with EoE was independent of sensitization. In addition to TSLP and the c11orf30 and STAT6 loci, which have previously been associated with allergic/inflammatory conditions by GWAS, we identified two loci that appear to be EoE specific. The chr19 locus which spans three genes, ANKRD27 , PDCD5 and RGS9BP and a locus at chr2p23.1 that spans the CAPN14 gene. CAPN14 has recently been reported to be associated with EoE following a meta-analysis of 736 samples [23] . The same study also reported associations at two additional loci at XKR6 and an intergenic region on 15q13, neither of these loci showed any evidence of association in our study (XKR6 rs2898261 P 0.663; 15q13 rs8041227 P 0.5686). Of the three genes at the chr19 locus, ANKRD27 (also referred to as Varp), appears to be the most likely candidate, it has been shown to regulate the trafficking of melanogenic enzymes to epidermal melanocytes [24] , interestingly, discoloration of the oesophagus has recently been reported in 90% of the EoE patients [25] . ANKRD27 has also recently been shown to act as a kinetic inhibitor of SNARE complex formations involving VAMP7 (ref. 26 ), which is involved in apical transport in epithelial cells [27] and wound healing [28] . CAPN14 is a member of the calpain family. Calpains are a family of intracellular Ca 2+ -regulated cysteine proteases that have been shown to function in diverse biological processes including the cell cycle, platelet aggregation and myoblast fusion through proteolytic cleavage of their substrates. Calpains include both ubiquitous and tissue-specific members [29] . CAPN14 shows highly specific expression and initial publications did not detect expression in any tissues tested [30] ; however, the test panels used appear to have not included oesophagus. Data from the GTEx project [31] and The Human Protein Atlas [32] both indicate that CAPN14 expression is limited to the oesophageal mucosa ( Fig. 2 ). Phylogenetically, CAPN14 is most closely related to calpain 13 and both are divergent from the remainder of the protein family. A recent evolutionary study of the calpain family indicates that CAPN14 has undergone persistent functional divergence during evolution [33] . Figure 2: CAPN14 is highly expressed in the oesophagus. Transcriptome-sequencing data from the GTEx project indicates CAPN14 is predominantly expressed in the oesophageal mucosa ( n =106). Each boxplot represents a measure of CAPN14 gene expression, plotted on the y axis for a given tissue, plotted on the x axis. The measure of expression used is reads per kilobase million (RPKM). The boxplot whiskers represent the data range across the 106 replicates, with the notch in the box representing the median expression value. Full size image The tissue specificity of calpains can result in tissue-specific disease phenotypes [34] ; mutations in CAPN3 , a muscle-specific large subunit [35] , result in limb-girdle muscular dystrophy, type 2A (LGMD2A) [36] . The expression of both CAPN8 and CAPN9 is predominantly restricted to the gastric surface mucus (pit) cells in the stomach. Neither gene has yet been implicated in human disease; however, mouse knockout models are susceptible to ethanol-induced gastric mucosal injury, implicating both in gastric mucosal defence from external stressors [37] . Not only does CAPN14 appear to be expressed exclusively in the oesophagus, our results also indicate CAPN14 is overexpressed in EoE oesophageal epithelial cells compared with controls, consistent with a gain of function. Similar results have also recently been published showing upregulation of CAPN14 in primary epithelial cells from EoE biopsies and organotypic cultures after IL-13 simulation [23] . CAPN14 has previously been implicated in allergy and inflammation, it has been shown to be unregulated by IL-4 stimulation [38] . In a recent study of an asthma mouse model, inhibition of calpain by calpeptin resulted in a marked improvement of the asthma phenotype, reversing airway hyper-responsiveness, reducing airway inflammation, bronchoalveolar lavage fluid eosinophilia, sub-epithelial fibrosis and the inflammatory cytokine profile, including IL-4, IL-5, IL-13, transforming growth factor-β1 and ova-specific immunoglobulin E [39] . Inhibition of CAPN14 activity may therefore constitute a potential therapy for the most debilitating aspect of EoE, oesophageal inflammation and remodelling. Samples The EoE discovery cohort consisted of 603 clinically confirmed EoE patients of European ancestry and 3637 matched controls. 529 samples were collected from five US sites, including Children's Hospital of Philadelphia (CHOP), UCSD, Northwestern, Stanford and UCSM, the mean age of these cases was 8.75 years. A further 74 samples were collected from AMC, mean age was 39.9. The replication cohort consisted of 333 cases and 675 controls of European ancestry. The mean age of the replication cohort cases was 8.4 s.d. years. All cases were biopsy proven with an eosinophils/hpf (400 × ) count of ≥24 on proton pump inhibitor therapy for at least 8 weeks. The majority of EoE subjects in both discovery and replication cohorts were male, making up to 73% in the discovery cohort and 75% in the replication cohort. Moreover, 70% of the discovery cohort and 72% of the replication cohort had asthma, allergic rhinitis or atopic dermatitis. The study was approved by the Institutional Review Board of the CHOP. Written informed consent for participation in the study was obtained from all participants and their parents or guardians. Genotyping The discovery samples were genotyped on either the Illumina HumanHap550, HH610 and the replication samples were genotyped on the Illumina HumanOmni Express-12v1 arrays at the Center for Applied Genomics at CHOP. Standard quality-control parameters were applied to the data set, samples with chip-wide genotyping failure rate ≪ 5% were excluded. SNPs with minor allele frequencies of ≪ 1%, genotyping failure rates of > 2% and Hardy–Weinberg P values ≪ 1 × 10 −6 were excluded from further analysis. Genetic ancestry was determined by computing principal components on the data set using smartpca, a part of the EIGENSTRAT package, on 100,000 random autosomal SNPs in linkage equilibrium. Samples were clustered into four Continental ancestry groups (Caucasian, African including admixed African–American, Asian and native American/admixed Hispanic) by K-means clustering using the kmeans package in R. Population stratification Smartpca eigenvectors were included as covariates in a logistic regression to control for population stratification as required. To determine the genomic inflation for each case–control set, we carried out an association analysis on the genotype data using plink before imputation. If genomic inflation exceeded 1.03, principal components were included as covariates in the post-imputation GWAS. Duplicate samples and cryptic relatedness Pairwise inflammatory bowel disease workup values were generated for all samples using the plink genome command. Inflammatory bowel disease workup was performed independently on the samples of Caucasian and African ancestry. A random sample from any pair with a PI_HAT value exceeding 0.3 was excluded from further analysis. Imputation Imputation of untyped markers (~39 M) was carried out using IMPUTE2 after prephasing with Shapeit. Each chromosome was prephased separately. To prevent chip-based batch effects due to differences in variant densities, each chip type was prephased and imputed separately. Reference phased cosmopolitan haplotypes and recombination rates were obtained from the 1000 genomes project (1000 Genomes Phase I integrated variant set b37 March 2012 release). Imputation was carried out in 5 Mb intervals using an effective population size of 20,000 as recommended. As a measure of the overall imputation accuracy we compared the concordance between the imputed and known genotypes in the subset of SNPs for which genotyping data was available. At a call threshold of 0.9, over 99% of the imputed genotypes were called and over 96% of those were concordant with the known genotypes. Post-imputation association analysis Statistical tests for association were carried out using the SNPTESTv2 package. Single marker analyses for the genome-wide data were carried out using linear regression taking genotype uncertainty introduced by the imputation into account. Call threshold was set at 0.9. SNPs with an info score below 0.8 were excluded from further analysis; the score is a measure of the observed information for the estimate of the allele frequencies at each imputed SNP, which is obtained by splitting the data into two components, observed and missing, the observed data likelihood is then integrated over the missing data. Combined P values across the individual data sets were generated using both fixed-effect and random-effect meta-analyses as implemented in the metal package for the fixed effects and the RE2 model in the METASOFT package for the random effects. Transcriptome sequencing mRNA libraries were constructed from primary oesophageal epithelial cells derived from nine cases (55% male and 44% female; mean age 11.6) and three controls (33% male and 66% female; mean age 12.1) using the Illumina TruSeq RNA Sample Preparation Kit v2, according to the manufacturer’s instructions with 12 unique-indexed adapters. Libraries were sequenced on an Illumina HiSeq 2000, generating 7.5 Gb 100 bp paired-end reads per sample. Transcripts were assembled, transcript abundances estimated and tested for differential expression between cases and controls using the cufflinks package. Pathway analysis Differentially expressed genes from the transcriptome-sequencing experiment were separated into two lists of up- or downregulated genes in the cases versus controls. Inclusion criteria included a statistically significant differential expression test ( P range 5 × 10 −5 to 0.0019) and a minimum two log2 fold change. Enrichment of KEGG pathways, GO-terms and functional categories (SP_PIR_KEYWORDS) was analyzed using DAVID ( http://david.abcc.ncifcrf.gov/ ). How to cite this article : Sleiman, P. M. A. et al. GWAS identifies four novel eosinophilic oesophagitis loci. Nat. Commun. 5:5593 doi: 10.1038/ncomms6593 (2014).